The landscape of kinase fusions in cancer Human cancer genomes harbour a variety of alterations leading to the deregulation of key pathways in tumour cells. The genomic characterization of tumours has uncovered numerous genes recurrently mutated, deleted or amplified, but gene fusions have not been characterized as extensively. Here we develop heuristics for reliably detecting gene fusion events in RNA-seq data and apply them to nearly 7,000 samples from The Cancer Genome Atlas. We thereby are able to discover several novel and recurrent fusions involving kinases. These findings have immediate clinical implications and expand the therapeutic options for cancer patients, as approved or exploratory drugs exist for many of these kinases. Kinases activated by gene fusions represent an important class of oncogenes associated with both hematopoietic malignancies and solid tumours. They are produced by translocations or other chromosomal rearrangements, and their protein products often represent ideal targets for the development of cancer drugs. For example, imatinib induces remission in leukaemia patients who are positive for BCR – ABL1 fusions. More recently, crizotinib and ceritinib have produced significant clinical benefit results in patients with lung carcinomas and mesenchymal tumours harbouring anaplastic lymphoma kinase ( ALK ) fusions [1] , [2] . Advances in massively parallel sequencing technologies have enabled the genomic characterization of large panels of tumours through the study of their DNA. While such studies have helped to identify numerous point mutations and small insertion/deletions in genes driving tumorigenesis, our understanding of the landscape of gene fusions in solid tumours is incomplete. There are now several thousand cancer transcriptomes, assessed through RNA-seq, publicly available. Here we describe a computational pipeline for the identification of gene fusions that we applied to the entire RNA-seq data set from The Cancer Genome Atlas (TCGA). We identify several novel and recurrent fusions involving kinases that very likely play a role in cancer. These discoveries not only go beyond augmenting our understanding of the genomic landscape of cancers, but they also have immediate implications for cancer diagnosis and therapy. Hallmarks of kinase fusions in solid tumours We first assembled a computational pipeline to collect evidence for all possible gene fusions and then focused our analyses on the fusions involving a kinase. Given the very large number of samples, we prioritized the sensitivity of the fusion detection pipeline (Methods) while retaining the ability to exclude false-positive calls by filtering out fusions present in normal samples as well as highly recurrent fusions that were detected by the algorithm at improbable frequencies. We then focused our detailed analysis exclusively on recurrent ( n ≥2 across all cancer types), putatively functional kinase fusions ( Supplementary Fig. 1 ). 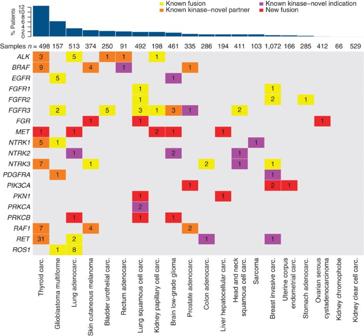Figure 1: Landscape of recurrent kinase fusions in solid tumours. Tumour types are indicated at the bottom and ordered by frequency of samples harbouring recurrent fusions (%; bar chart at the top). For each gene, the number of fusions found in TCGA samples is displayed in the matrix and coloured by the type of novelty. Yellow denotes kinase fusions that have been described previously in this particular indication; orange denotes kinase fusions for which one or more partner genes are novel but the indication is not; purple denotes a novel indication for a particular kinase fusion regardless of the identity of the partner gene; red denotes novel, recurrent kinase fusions. We comprehensively surveyed gene fusions across 20 solid tumour types ( Supplementary Table 1 , Supplementary Data 1 ) and identified several broad contours within the landscape of kinase fusions ( Fig. 1 ). First, as has been observed for point mutations, the proportion of samples harbouring kinase fusions was markedly different between cancer types, reflecting differences in the aetiology of these tumours. For instance, sarcoma samples showed the highest frequency of kinase fusions (0.57 fusions per sample), consistent with the current understanding that a large fraction of sarcomas harbour specific translocations, but only 12% of those were recurrent kinase fusions ( Supplementary Fig. 1 ). Other tumour types, including thyroid cancer and glioblastoma, showed a lower frequency of kinase fusions on average (0.19 and 0.23 fusions per sample, respectively) but a relatively high proportion of these were recurrent fusions (67% and 36%, respectively), suggesting a more prominent role of kinase fusions in these cancers. Conversely, some cancer types, for example, clear cell and chromophobe renal cell carcinoma, showed a very low frequency of kinase fusions with no instances of recurrence ( Supplementary Fig. 1 ). Overall, we detected recurrent kinase fusions in 3.0% of the samples, and all cancers except clear cell and chromophobe renal cell carcinoma harboured recurrent kinase fusions (0–12.9% of samples per cancer type, median=2.1%). Figure 1: Landscape of recurrent kinase fusions in solid tumours. Tumour types are indicated at the bottom and ordered by frequency of samples harbouring recurrent fusions (%; bar chart at the top). For each gene, the number of fusions found in TCGA samples is displayed in the matrix and coloured by the type of novelty. Yellow denotes kinase fusions that have been described previously in this particular indication; orange denotes kinase fusions for which one or more partner genes are novel but the indication is not; purple denotes a novel indication for a particular kinase fusion regardless of the identity of the partner gene; red denotes novel, recurrent kinase fusions. Full size image Second, our pipeline was able to recapitulate most known translocation events in cancer ( ALK , BRAF , EGFR , FGFR1 , 2 and 3 , NTRK1 , 2 and 3 , PDGFRA , PRKCA , RAF1 , RET , ROS1 ). Interestingly, we identified new tumour types harbouring such fusions and discovered several novel fusion partners for these kinases. We also detected several low-frequency, pan-cancer kinase fusion events, for example in the neurotrophic tyrosine receptor kinases NTRK1 , NTRK2 and NTRK3 , that drive tumorigenesis in a small fraction of multiple cancers, regardless of tissue type ( Fig. 1 ). Third, we identified several novel and recurrent kinase fusions that very likely play a role in cancer, such as those involving the MET proto-oncogene and PIK3CA (phosphatidylinositol-4,5-bisphosphate 3-kinase, catalytic subunit alpha). These bona fide oncogenes have not been shown previously to be activated by fusion events. Our analysis also uncovered novel, recurrent fusions in kinases with no known tumorigenic genomic alterations (that is, feline Gardner–Rasheed sarcoma viral oncogene homologue, FGR and protein kinase N1, PKN1 ), potentially resulting in active and oncogenic fusion proteins. Finally, we discovered a recurrent fusion in sarcoma encoding the non-catalytic portion of TRIO kinase, which resulted in the upregulation of the transcription of telomerase reverse transcriptase ( TERT ) in those tumours. Kinases known to be involved in gene fusions ALK fusions, including EML4 – ALK , TFG – ALK and STRN – ALK , have been identified in multiple cancer types, including lung adenocarcinoma [3] , colorectal [4] , breast [5] , renal cell [6] , renal medullary [7] and thyroid cancers [8] . Consistent with previous studies, we detected EML4 – ALK fusions in ~1% (5/513) of lung adenocarcinoma samples, multiple ALK fusions, including a single STRN – ALK fusion, in thyroid cancer (3/498) and one in papillary renal carcinoma. We also found several novel ALK fusion events, including a TPM1 – ALK fusion in bladder cancer, a SMEK2 – ALK fusion in rectal adenocarcinoma and a GTF2IRD1 – ALK fusion in thyroid cancer ( Fig. 1 , Supplementary Fig. 2 ), adding weight to the emerging notion that known driver events in certain tumours can also play a role in other tumour types, regardless of histology. We also identified multiple c-ros oncogene 1 ( ROS1 ) fusions, including ROS1 fusions in 8/513 lung adenocarcinomas, all of which have been previously described [9] , [10] , [11] , [12] . In addition, we detected a CEP85L – ROS1 fusion in a glioblastoma tumour sample ( Fig. 1 , Supplementary Fig. 3 ). A similar fusion was recently reported in a single angiosarcoma sample [13] . RET proto-oncogene fusions have been identified previously in both lung adenocarcinoma [4] , [14] and thyroid cancer [15] . Consistent with these studies, we observed recurrent CCDC6 – RET fusions in thyroid cancer [15] but also identified several RET fusions with novel partners, including AKAP13 , FKBP15 , SPECC1L and TBL1XR1 ( Fig. 1 , Supplementary Fig. 4 ). Three of these 5′ fusion partners contain dimerization-competent coiled-coil motifs within the coding region, while the fourth, TBL1XR1, contains a LisH (Lis-homology) motif, which is similarly capable of dimerization [16] and therefore likely leading to RET activation. In addition, we detected previously identified RET fusions in new tumour indications, including a single CCDC6 – RET fusion in colon adenocarcinoma and a single ERC1 – RET fusion in breast cancer. In total, we observed RET fusions in four of the 20 cancer types analysed, providing a therapeutic rationale for the use of RET inhibitors in multiple patient subpopulations. BRAF (v-raf murine sarcoma viral oncogene homologue B) fusions have also been described previously in multiple cancer types, including prostate cancer [17] , melanoma [18] , radiation-induced thyroid cancer [19] and pediatric low-grade gliomas [20] . Consistent with these studies, we identified a broad range of cancer types harbouring BRAF fusions, including prostate, melanoma and thyroid. We also detected a single TRIM24 – BRAF fusion in rectal adenocarcinoma. Interestingly, the BRAF fusions in melanoma are exclusive of other known oncogenic events such as BRAF and NRAS mutations. Many of the specific fusions we report here, including AGK – BRAF [19] , SND1 – BRAF [21] , MACF1 – BRAF [20] , TAX1BP1 – BRAF and CDC27 – BRAF [18] , have been previously identified. A number of BRAF fusions are, however, novel ( Fig. 1 , Supplementary Fig. 5 ), including ATG7 – BRAF in melanoma, as well as ZC3HAV1 – BRAF and FAM114A2 – BRAF in thyroid cancer. These three fusions encode 5′ protein partners that contribute coiled-coil (CC) or zinc-finger dimerization motifs, which likely produce constitutively activated BRAF dimers capable of driving tumorigenesis and poorly sensitive to RAF inhibitors, but sensitive to inhibition downstream, through MEK (mitogen-activated protein kinase kinase 1 and 2) inhibition for instance [18] . Other novel BRAF fusions identified do not encode protein partners with obvious dimerization motifs. However, these fusions all remove at least the first eight exons of BRAF, which has previously been shown to promote BRAF dimerization, independent of activated RAS (rat sarcoma viral oncogene homologues) or other mechanisms of BRAF dimerization [22] . These fusions similarly seem capable of promoting tumorigenesis. Consistent with previous studies [17] , [23] , we also found recurrent RAF1 (also known as CRAF ) fusions in various tumour types ( Fig. 1 , Supplementary Fig. 6 ). In addition to known tumour occurrences (four fusions in melanoma, two fusions in prostate adenocarcinoma), we identified AGGF1 – RAF1 fusions in seven papillary thyroid carcinoma samples (1.4%). This is remarkable not only because RAF1 fusions have never been identified in this cancer type before, but also because all seven examples involved a novel partner gene, AGGF1 ( angiogenic factor with G patch and FHA domains 1 ). AGGF1 contains an N-terminal coiled–coil dimerization motif likely to activate RAF1 in a fashion similar to BRAF fusions, by forming constitutively activated, RAF inhibitor resistant, RAF1 dimers. AGGF1 – RAF1 fusions appear not to be limited to thyroid cancers, as we also found a single AGGF1 – RAF1 fusion in prostate cancer. We observed a broad distribution of the fibroblast growth factor receptors FGFR1 , FGFR2 and FGFR3 fusions—in particular FGFR3 – TACC3 fusions—across eight of the 20 tumour types analysed ( Fig. 1 ). This is consistent with recent studies, which identified recurrent FGFR family fusions in multiple cancer types [24] , [25] . We also detected a single FGFR3 – TACC3 fusion in a novel indication, papillary renal carcinoma, and a novel FGFR3 – ELAVL3 fusion in low-grade glioma ( Supplementary Fig. 7 ). Similar to RET and NTRK1 – 3 (see below), fusions involving FGFR1 – 3 provide a therapeutic opportunity for current and future FGFR inhibitors in multiple patient subpopulations. Recurrent fusions involving members of the NTRK family have been identified previously in congenital fibrosarcoma [26] , human secretory breast carcinoma [27] and papillary thyroid cancer [28] , which represent clinical indications for which currently available non-kinase-targeted treatment options are usually adequate. However, recurrent NTRK1 and NTRK2 fusions have also been recently identified in diseases which represent significant unmet medical needs, including glioblastoma [29] , cholangiocarcinoma [30] and pediatric high-grade glioma [24] . Consistent with previous studies, we observed recurrent NTRK1 and NTRK3 fusions in papillary thyroid cancer and glioblastoma, but also identified a number of novel NTRK2 fusions in head and neck squamous cell carcinoma ( PAN3 – NTRK2 ), low-grade glioma ( AFAP1 – NTRK2 ) and lung adenocarcinoma ( TRIM24 – NTRK2 ) ( Fig. 1 , Supplementary Fig. 8 ). In addition, we observed a known NTRK1 fusion ( TPM3 – NTRK1 ) in sarcoma, previously described only in thyroid cancer [31] . Across all tumour types analysed, NTRK1–3 fusions were observed at low frequency in 9 of the 20 cancer types analysed, providing a therapeutic opportunity for the use of pan-NTRK inhibitors in multiple patient populations. Protein kinase C fusions have recently been described in papillary glioneuronal tumours [32] and benign fibrous histiocytoma [33] . We found two new occurrences of PRKCA (protein kinase C, alpha) fusions in lung squamous cell carcinoma and three PRKCB (protein kinase C, beta) fusions in lung squamous cell carcinoma, lung adenocarcinoma and low-grade glioma ( Fig. 1 , Supplementary Fig. 9a,c ). In one instance, PRKCA was fused with IGF2BP3 (insulin-like growth factor 2 messenger RNA ( mRNA ) binding protein 3), an mRNA binding protein present in the nucleus and the cytoplasm. The functional domains of IGF2BP3, such as a nucleotide binding/RNA recognition domain, are intact in the fusion; however their contribution to PRKCA activation is unclear. The second fusion, TANC2 – PRKCA , encodes only the first two exons of TANC2 (tetratricopeptide repeat, ankyrin repeat and CC containing 2), which contain no annotated structural domain or motif. In both cases, however, N-terminal truncation of PRKCA removes the autoinhibitory pseudosubstrate segment, possibly leading to a constitutively activated kinase in the absence of a functional fusion partner. In addition, we noticed a tendency towards overexpression of PRKCA in these two fusion-harbouring samples ( PRKCA mRNA expression z -scores: 6.8 and 2.6 in the samples harbouring the TANC2 – PRKCA and IGF2BP3 – PRKCA fusions, respectively; Supplementary Fig. 9b ). These data suggest that PRKCA fusions are potential oncogenic events in lung squamous cell carcinoma, leading to overexpression as well as constitutive activation of PRKCA. In the same fashion, PRKCB fusions truncate the N-terminal part of the protein containing the autoinhibitory domain and are predicted to activate this kinase ( Supplementary Fig. 9c ). Taken together, these data suggest an emerging critical role for protein kinase C alpha and beta in the tumorigenesis of non-small cell lung cancer. Novel fusions involving known oncogenes The MET proto-oncogene is implicated in a variety of cancers, particularly in papillary renal cell carcinoma where a number of somatic mutations have been described [34] . Anecdotally, a transforming TPR – MET fusion was previously generated in vitro via carcinogen-induced chromosomal rearrangement fusing the dimerization domain of TPR to the kinase domain of the MET receptor tyrosine kinase [35] . Here, we report for the first time in primary tumour samples recurrent translocation events involving MET . Two in-frame MET fusions in papillary renal carcinoma, BAIAP2L1 – MET and C8orf34 – MET, were detected with predicted protein products containing amino-terminal dimerization domains fused to the intracellular domain of MET. BAIAP2L1 contains a CC region while C8orf34 contains a regulatory subunit of cAMP-dependent protein kinase, both of which act as dimerization motifs ( Fig. 2 ). Notably, BAIAP2L1 was recently described as a 3′ fusion partner for FGFR3 in bladder cancer [36] , incorporating the same CC region as the 5′ fusion described here. We also identified single MET fusions in four other cancers: low-grade glioma, hepatocellular carcinoma, lung adenocarcinoma and thyroid carcinoma. In at least two out of these four cases ( KIF5B – MET in lung adenocarcinoma and TFG – MET in thyroid papillary carcinoma), the predicted chimeric protein follows the classic activation paradigm, fusing dimerization motifs to an intact kinase domain. These results are remarkable because MET is a known oncogene that has not previously been implicated in translocation events. This mechanism could account for a significant fraction of total MET oncogenic activation events and therefore represents druggable intervention opportunities for patients with these tumours. 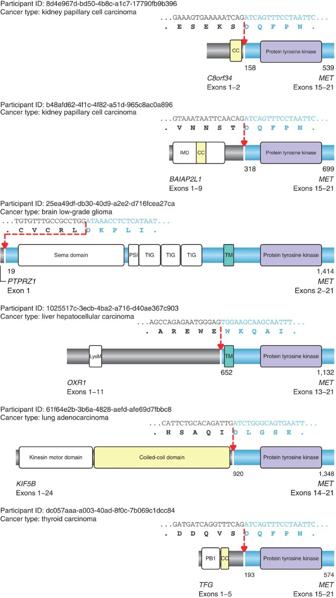Figure 2: Structural details ofMETfusions. Novel fusions ofMETproto-oncogene in five cancer types. Protein domains, sample details, cancer type, gene partners, as well as genomic and amino-acid sequence are indicated for each of the six predictedMETkinase fusion proteins. In addition, the protein coordinates of the fusion breakpoints and the total amino-acid length of the fusion protein are noted under each protein structure. The protein tyrosine kinase domains are coloured in purple, the transmembrane domains (TM) are indicated in teal, CC dimerization domains are indicated in yellow, whereas other domains are left in white. Fusion breakpoints are delineated by red arrows. IMD, IRSp53/MIM homology domain; PSI, Plexin repeat domain; TIG, IPT/TIG immunoglobulin-like domain; LysM, lysin motif domain; PB1, Phox and Bem1p domain. Figure 2: Structural details of MET fusions. Novel fusions of MET proto-oncogene in five cancer types. Protein domains, sample details, cancer type, gene partners, as well as genomic and amino-acid sequence are indicated for each of the six predicted MET kinase fusion proteins. In addition, the protein coordinates of the fusion breakpoints and the total amino-acid length of the fusion protein are noted under each protein structure. The protein tyrosine kinase domains are coloured in purple, the transmembrane domains (TM) are indicated in teal, CC dimerization domains are indicated in yellow, whereas other domains are left in white. Fusion breakpoints are delineated by red arrows. IMD, IRSp53/MIM homology domain; PSI, Plexin repeat domain; TIG, IPT/TIG immunoglobulin-like domain; LysM, lysin motif domain; PB1, Phox and Bem1p domain. Full size image Mutations and, to a lesser extent, increased copy numbers in another prevalent oncogene, PIK3CA , have been characterized in diverse cancers. While activating missense mutations in PIK3CA have been described as frequently as 50% in endometrial cancers, 30% in breast invasive carcinomas and 20% in colorectal as well as head and neck cancers [37] , this gene has not been implicated in activating fusion events. We found two TBL1XR1 – PIK3CA fusions in 1,072 breast cancer samples, and a single occurrence of the same gene fusion in prostate adenocarcinoma (1/335). In addition, one FNDC3B – PIK3CA fusion was found in uterine corpus endometrial carcinoma (1/166) ( Fig. 1 , Supplementary Figs 10 and 11 ). The nucleotide sequence of the fusion transcripts suggested that the complete wild-type sequence of PIK3CA was expressed in all four cases, with the partner gene contributing only the 5′UTR (untranslated region), and thereby driving overexpression of PIK3CA ( Fig. 3a ). Indeed, in all samples where we detected PIK3CA translocations, and where PIK3CA was not amplified, PIK3CA mRNA expression levels were the highest within the respective tumour types ( Fig. 3b–d ). Interestingly, TBL1XR1 is thought to regulate the expression of nuclear hormone receptor co-repressors [38] , and both tissue types in which TBL1XR1 – PIK3CA fusions were found (invasive breast carcinoma and prostate cancer), are hormone driven and ranked among the highest for TBL1XR1 mRNA expression across all normal tissues ( Supplementary Fig. 12 ). These results strongly suggest that PIK3CA overexpression is driven by its fusion partner, and that PIK3CA promoter fusions are an additional oncogenic mechanism to be considered for expanding the use of targeted therapies such as PI3K, AKT or mTOR inhibitors. 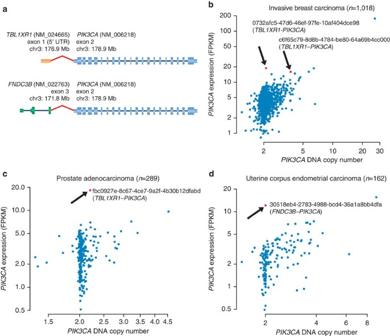Figure 3:PIK3CApromoter fusions. Novel fusions ofPIK3CAin three cancer types. (a) Genomic structure ofTBL1XR1–PIK3CAandFNDC3B–PIK3CAfusions. In both cases, the entire coding sequence ofPIK3CAis present in the predicted fusion sequence. RefSeq IDs, exon numbers and genomic coordinates are indicated. Exon 1 ofTBL1XR1(5′UTR) is fused to exon 2 ofPIK3CA(5′UTR). In the case ofFNDC3B–PIK3CA, exon 3 ofFNDC3Bis fused to the 5′UTR ofPIK3CA. (b–d) Scatter plots ofPIK3CADNA copy number versus mRNA expression across all TCGA samples for which both data types are available. Samples harbouring aPIK3CAfusion are depicted in red (along with TCGA sample ID) and show a high expression ofPIK3CArelative to the other samples. FPKM, fragments per kilobase of transcript per million mapped reads. Figure 3: PIK3CA promoter fusions. Novel fusions of PIK3CA in three cancer types. ( a ) Genomic structure of TBL1XR1 – PIK3CA and FNDC3B – PIK3CA fusions. In both cases, the entire coding sequence of PIK3CA is present in the predicted fusion sequence. RefSeq IDs, exon numbers and genomic coordinates are indicated. Exon 1 of TBL1XR1 (5′UTR) is fused to exon 2 of PIK3CA (5′UTR). In the case of FNDC3B – PIK3CA , exon 3 of FNDC3B is fused to the 5′UTR of PIK3CA . ( b – d ) Scatter plots of PIK3CA DNA copy number versus mRNA expression across all TCGA samples for which both data types are available. Samples harbouring a PIK3CA fusion are depicted in red (along with TCGA sample ID) and show a high expression of PIK3CA relative to the other samples. FPKM, fragments per kilobase of transcript per million mapped reads. Full size image Novel recurrent fusions In addition to fusions involving known oncogenes, we found several novel and recurrent fusions involving kinases that have not been previously directly linked to cancer ( Fig. 1 , Supplementary Data 2 ). One of these kinases was FGR , a member of the Src family of protein tyrosine kinases. Here, we show for the first time that genetic events can lead to FGR overexpression in primary tumour samples. We found three WASF2 – FGR fusions (in lung squamous carcinoma, ovarian serous cystadenocarcinoma and skin cutaneous melanoma), harbouring the exact same breakpoints in all cases ( Supplementary Figs 13 and 14 ). The WASF2 and FGR genes are located very proximally on the short arm of chromosome 1, and the fusion presumably results from a tandem repeat that puts their coding regions in close proximity ( Supplementary Fig. 15a,b ). Somewhat similarly to TBL1XR1 – PIK3CA , the promoter and 5′UTR of WASF2 are fused with the 5′UTR of FGR , leading to mis- or overexpression of the entire wild-type sequence of the protein. In all three cases, FGR mRNA expression in the samples harbouring a fusion was among the highest compared with all other tumours of that tissue type ( Supplementary Fig. 15c–e ). Even though FGR has not been genetically linked to cancer to date, it has been hypothesized that its expression could compensate for SRC inhibition [39] . Collectively, these data highlight a previously undocumented mechanism of genetic deregulation of a Src family member. PKN1 has been implicated in androgen-associated prostate carcinomas [40] and in Wnt/β-catenin signalling in melanomas [41] . We detected fusions of PKN1 in samples of squamous cell carcinoma of the lung and hepatocellular carcinoma ( Fig. 1 , Supplementary Fig. 16a ). mRNA expression levels of both fusions are high within the respective tumour types ( Supplementary Fig. 16b,c ). Interestingly, the protein sequences contributed by the non-kinase fusion partners were very limited in both cases (three and five amino acids in ANXA4 – PKN1 and TECR – PKN1 , respectively) and resulted in a truncated PKN1 protein product missing the PKN1 N terminus. This is notable because this protein region contains regulatory domains that suppress kinase activity in the absence of binding to Rho-GTP [42] . PKN1 also has a Caspase-3 cleavage site near the breakpoint of both fusions that normally results in activation of the kinase on cleavage [43] ( Supplementary Fig. 16a ). Therefore, both of these fusions are potentially activating in the absence of any functional or structural contribution from the non-kinase fusion partners. It is attractive to speculate that both fusion events cause increased PKN1 expression and constitutive activation of the kinase, leading to enhanced cell proliferation. We describe here a pan-cancer analysis of the transcriptomes of nearly 7,000 tumours from TCGA that is specifically focused on kinase gene fusion events. Overall, 3.0% of tumour samples contained a likely oncogenic, recurrent kinase fusion (2.1% excluding thyroid cancer). The observed striking differences in the frequencies of kinase fusions across solid tumours are consistent with previous data on the relative contributions of diverse types of genetic aberrations to tumourigenesis. Certain tumour types, such as ovarian serous carcinoma, harbour a large number of somatic copy number alterations, but exhibit a relatively simple mutational profile [44] . Other tumour types such as melanoma carry predominantly somatic point mutations [45] . Consistent with these observations, our data suggest that certain cancers are heavily driven by kinase rearrangements. Notably, thyroid cancers have the highest frequency of recurrent kinase fusions (63/498, 13%), and all fusion events including ALK , BRAF , MET , NTRK1 , NTRK2 , RAF1 and RET are mutually exclusive in this cancer type ( Fig. 4 ). These data provide a strong genetic rationale that these alterations are driver events. In stark contrast, clear cell and chromophobe renal cell carcinoma have the lowest frequencies of kinase fusions, none of which were recurrent in our analysis of this data set ( Supplementary Fig. 1 ). 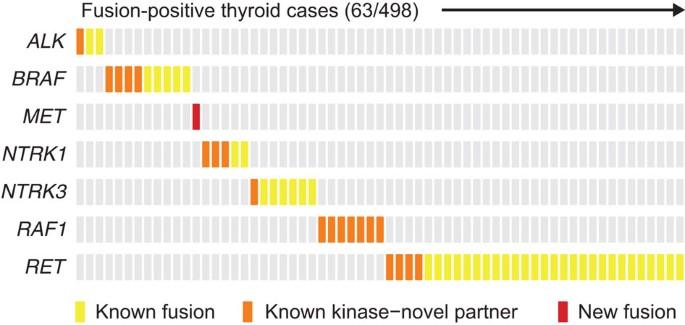Figure 4: Mutual exclusivity of fusions in thyroid cancer. All samples harbouring a recurrent kinase fusion in any of the genes indicated on the left are displayed on thexaxis. The type of fusion is depicted as a coloured box with the same color-coding scheme as inFig. 1. Yellow denotes kinase fusions that have been described previously in thyroid cancer; orange denotes kinase fusions in which the partner gene is novel; red denotes novel recurrent kinase fusions. In all cases, the presence of a kinase fusion is exclusive of any other fusion involving kinases recurrently fused. Figure 4: Mutual exclusivity of fusions in thyroid cancer. All samples harbouring a recurrent kinase fusion in any of the genes indicated on the left are displayed on the x axis. The type of fusion is depicted as a coloured box with the same color-coding scheme as in Fig. 1 . Yellow denotes kinase fusions that have been described previously in thyroid cancer; orange denotes kinase fusions in which the partner gene is novel; red denotes novel recurrent kinase fusions. In all cases, the presence of a kinase fusion is exclusive of any other fusion involving kinases recurrently fused. Full size image Our study primarily aimed to identify recurrent, potentially oncogenic fusions involving kinases. In addition to rediscovering previously known recurrent kinase fusions, we identified new fusion partners for many genes (for example, TPM1 – ALK in bladder cancer, TBL1XR1 – RET in thyroid cancer, and so on). Our study also revealed new cancer types harbouring known fusions (for example, BRAF fusion in rectal adenocarcinoma, FGFR3 fusion in prostate adenocarcinoma, RET fusions in colon adenocarcinoma and invasive breast carcinoma, EGFR – SEPT14 in low-grade glioma, and so on). These discoveries not only go beyond simply augmenting our understanding of the genomic landscape of cancers, but they also have immediate implications for cancer diagnosis and therapy. First, our new findings justify a rapid reassessment of current protocols for targeted genomic profiling of patients, which are insufficient to detect these aberrancies, to cover therapeutically actionable fusion events across cancers. In addition, our findings will hopefully motivate both industrial and academic investigators interested in drug discovery to engage in the development of cancer drugs against targets that have not been considered previously because they might have represented an insufficient fraction of targetable events. Along these lines, our pan-cancer analysis revealed that although certain kinase fusions only occurred once within a tumour type, they are clearly recurrent when multiple tissue types are considered, supporting the emergence of innovative clinical trial designs such as the ‘basket’ trials. For example, we found six cancer types with a single fusion in a gene of the NTRK family, but altogether, we detected a total of 23 NTRK1 , NTRK2 and NTRK3 fusions across nine tumour types. These data strongly suggest that gene fusions are one of the most prevalent mechanisms of oncogenic activation of this receptor tyrosine kinase family. NTRK fusions therefore represent a low frequency, pan-cancer event that nevertheless may account for a significant fraction of patients who could benefit from a pan-NTRK inhibitor. Notably, this analysis uncovered several new aberrations that may drive tumourigenesis through constitutive activation of a kinase due to a fusion event. In particular, we found recurrent fusions of MET and PIK3CA that are both bona fide oncogenes commonly activated by gene amplification or point mutations. The activation of MET by fusion with a partner gene is most likely due to constitutive dimerization of the receptor. In contrast, TBL1XR1 – PIK3CA fusions likely drive increased PIK3CA mRNA expression by juxtaposing the promoter region of the partner gene to the 5′ end of the intact PIK3CA coding sequence. Another example of such ‘promoter fusions’ is the recurrent WASF2 – FGR fusion, which we found in three cancer types. We also observed fusions in some Ser/Thr kinases (for example, PRKCA , PKN1 ), where deletion of their regulatory N-terminal domain putatively leads to constitutive activation by de-repression of the kinase activity. Additional studies, expanding on our analyses, are necessary to uncover the mechanistic details of these newly described fusions and to further validate biologically the hypotheses we have put forward here. Given the number of samples that we analysed (nearly 7,000 samples across 20 tumour types) and the observed frequencies of kinase fusion events across solid tumours, relatively few kinases appear to be recurrently fused in-frame with another gene while conserving an intact kinase domain ( Supplementary Fig. 1 ). Therefore, a pure frequency threshold (that is, recurrence) allowed us to identify several new kinase fusion driver candidates. By excluding all kinases that were involved in only one fusion event across the entire data set, we disregarded several singletons that passed all other filtering criteria and showed the characteristics of functional fusions. With increasing numbers of tumours and additional cancer types being sequenced in the future, it is probable that some of these kinase fusions will appear more frequently and prove to be important drivers. One such example is PRKACA (protein kinase, cAMP -dependent, catalytic, alpha), which was recently shown to be fused in 100% (15/15) of fibrolamellar hepatocellular carcinoma [46] . Only one sample of fibrolamellar hepatocellular carcinoma was included in the TCGA data set that we analysed, and our study revealed that it indeed harboured the characteristic DNAJB1 – PRKACA fusion. However, the majority of singleton gene fusions in this set are predicted to be passenger events, occurring as a consequence of chromothripsis or genomic instability. In addition, focal events such as gene amplification also contribute passenger events. This is likely the case for ERBB2 , PAK1 , PDGFRA and RPS6KB1 ( Supplementary Data 2 and 3 ) [47] . Finally, we predict that eventually some important, biologically meaningful fusions will be discovered that involve the non-enzymatic portion of kinases as partner genes. Although not the focus of this study, we describe here such an example: a recurrent fusion in two dedifferentiated liposarcoma samples (2/38; 5%) encoding the non-kinase portion of TRIO , which results in upregulation of its fusion partner TERT ( Fig. 5a,b ). Telomerase activity is a hallmark of many cancers, and two other genetic mechanisms of TERT reactivation have been described recently; both somatic mutations in the promoter of the TERT gene [48] and DNA copy number gains of TERT [49] were shown to activate its transcription. We observed that the two liposarcoma samples harbouring TRIO – TERT fusions display a TERT mRNA expression level ~100-fold higher than measured in samples without such a fusion. These findings raise the possibility that TERT fusions might represent an alternative mechanism for telomerase reactivation in cancers. 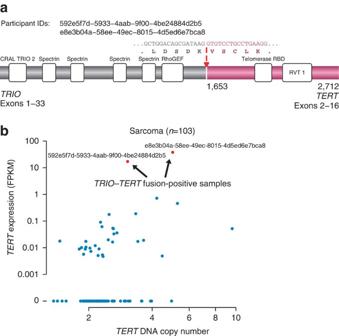Figure 5: NovelTRIO–TERTfusions in liposarcoma samples. (a) Protein domains as well as genomic and amino-acid sequences are indicated for theTRIO–TERTfusion protein. Protein coordinates of the fusion breakpoints and the total amino-acid length of the fusion protein are noted under the protein structure; fusion breakpoint is delineated by a red arrow. CRAL TRIO 2, divergent CRAL/TRIO domain; Telomerase RBD, telomerase ribonucleoprotein complex–RNA binding domain; RVT 1: reverse transcriptase (RNA-dependent DNA polymerase). (b) Scatter plot ofTERTDNA copy number versus mRNA expression across all TCGA samples for which both data types are available. Samples harbouring aTERTfusion are depicted in red (along with TCGA sample ID) and show a high expression ofTERTrelative to the other samples. FPKM: Fragments per kilobase of transcript per million mapped reads. Figure 5: Novel TRIO – TERT fusions in liposarcoma samples. ( a ) Protein domains as well as genomic and amino-acid sequences are indicated for the TRIO – TERT fusion protein. Protein coordinates of the fusion breakpoints and the total amino-acid length of the fusion protein are noted under the protein structure; fusion breakpoint is delineated by a red arrow. CRAL TRIO 2, divergent CRAL/TRIO domain; Telomerase RBD, telomerase ribonucleoprotein complex–RNA binding domain; RVT 1: reverse transcriptase (RNA-dependent DNA polymerase). ( b ) Scatter plot of TERT DNA copy number versus mRNA expression across all TCGA samples for which both data types are available. Samples harbouring a TERT fusion are depicted in red (along with TCGA sample ID) and show a high expression of TERT relative to the other samples. FPKM: Fragments per kilobase of transcript per million mapped reads. Full size image Overview Briefly, fusions between any two genes were identified based on the number of chimeric reads (sequencing paired ends mapping to different genes) and split reads (spanning a fusion breakpoint), concordance between the strands of the reads and the genes involved in the putative fusion, and a number of filtering criteria to flag false positive and non-functional fusions. In addition, recurrent kinase fusions observed in a panel of 600 normal samples from TCGA and 1,800 normal samples from the Genotype–Tissue Expression (GTEx) project were also excluded from further analysis. Finally, all recurrent kinase fusions ( n ≥2) were manually reviewed to identify putative oncogenic drivers with distinctive characteristics of functional kinase fusions. In particular, the following features were required: presence of an intergenic junction between two exons, a predicted in-frame coding sequence and conservation of the complete kinase catalytic domain. Conversely, we excluded false positives from further analysis according to two main criteria: the presence of a homologous or repetitive sequence shared by the two fusion partners causing an alignment artifact, or the very high expression of one or both fusion partners. Origin of data To comprehensively identify the landscape of kinase fusions in solid tumours, we analysed RNA-seq data from 20 solid tumour types in TCGA (6,893 samples, Supplementary Table 1 and Supplementary Data 1 ), including provisional TCGA data from sarcoma tumours (103 samples). All available unaligned RNA-seq data files (fastq files) were obtained from the Cancer Genomics Hub (CGHub) and loaded into our processing pipeline. In addition, the clinical data from all available tumour types were pulled from the TCGA FTP server ( https://tcga-data.nci.nih.gov/tcgafiles/ftp_auth/distro_ftpusers/anonymous/tumour ). Fusion detection algorithm and filtering Using the STAR v2.3.1q aligner [50] , RNA-seq data from each tumour sample was aligned to version hg19 of the human genome, while also providing transcriptome and splice junction annotations from the Gencode project v17 (ref. 51 ). A different genome index was generated for each of the different read lengths encountered in the RNA-seq data. Runtime options passed to STAR to generate genome indexes included: STAR --runMode genomeGenerate, --genomeDir hg19_Gencode17.overhang<read-length>, --genomeFastaFiles <hg19 reference fasta files>, --sjdbGTFfile gencode.annotation.gtf and --sjdbOverhang <read-length–1>. STAR was then used to produce alignments and was run with specific options including: STAR --readFilesIn <fastq_1.fq.gz> <fastq_2.fq.gz>, --readFilesCommand zcat, --genomeDir <STAR genome index>, --outSAMstrandField intronMotif, --outFilterIntronMotifs RemoveNoncanonicalUnannotated, --outReadsUnmapped None, --chimSegmentMin 15, --chimJunctionOverhangMin 15, --alignMatesGapMax 200000 and --alignIntronMax 200000. Given the programme arguments described above, the output of the STAR aligner consisted of two separate files containing sequencing reads: aligned reads consistent with a normal reference (_Aligned.sam) and aligned reads indicative of a putative rearrangement (_Chimeric.sam). A fusion detection routine was then used to identify protein fusion candidates: using the python library HTSeq-0.5.4p1 (ref. 52 ) and transcriptome annotations from the Gencode project v17, the name-sorted ‘chimeric’ alignments in the output of the STAR aligner were examined to count the number of chimeric pairs (where each sequencing end aligns to a different gene) and reads split between two genes. Specific filters were then applied to improve specificity: the strands of the alignments were compared with the strands of the genes to keep only those consistent with a proper 5′→3′ fusion; putative fusions between homologous genes were discarded; putative fusions between genes and overlapping homologous genes were discarded as well. This procedure then returned the complete list of possible gene fusions in a given sample, modulo the alignment artifacts, along with the number of chimeric reads and split reads supporting each fusion. Next, fusions were filtered based on the number of chimeric reads and paired reads supporting them: five chimeric reads or more were required when two or more split reads were present; 10 chimeric reads or more were required when only 1 split read was present; 20 chimeric reads or more were required when no split reads were detected. Finally, the output of the fusion detection step above was filtered to further improve specificity. This step relied on the analysis of a large number of samples to filter out highly recurrent fusions that were detected at improbable frequencies within a cancer type: for instance, fusions detected in >95% of samples, or fusions where both gene partners are themselves involved in >1 fusions in >25% of samples, were flagged as putative false positives. In addition, recurrent kinase fusions observed using the same procedure in five samples or more in a panel of 647 normal samples from TCGA (downloaded from CGHub on 2014-03-10) and 1,750 normal samples from the GTEx project (downloaded from dbGaP project phs000424.v4.p1 on 2014-01-17, excluding all transformed and cancer cell lines) were also excluded. This allowed us to exclude a large number of library construction and alignment artifacts. All recurrent kinase fusion candidates ( n ≥2 across cancer types) identified by this procedure were then manually reviewed in the Integrative Genomics Viewer [53] to identify putative drivers with distinctive patterns of functional kinase fusions, and reject passenger and false-positive fusions. In particular, the following features were required for putative functional fusions: (1) presence of an intergenic junction (between two exons or between an exon and a cryptic exon); (2) a predicted in-frame coding sequence; (3) conservation of the full kinase catalytic domain. Manual review was facilitated by the fact that passenger fusions could mainly be linked to the following: (1) the absence of a fusion protein coding sequence that was in-frame; (2) the kinase domain was absent or truncated from the predicted protein sequence; or (3) the kinase was found to be fused only once in all samples (non-recurrent fusion). Conversely, we flagged false positives according to two main causes: (1) a homologous or repetitive sequence shared by the two fusion partners and causing an alignment artifact, or (2) very high expression of one or both fusion partners in a particular sample, causing the production of non-specific RNA chimera by trans -splicing. This process, occurring at the step of cDNA preparation through template switching by the reverse transcriptase [54] , produces multiple experimental artifacts that can appear like real fusions but lack a clear exon–exon breakpoint and generally are not supported by split reads. Functional annotation Recurrent candidate fusion protein sequences were searched for structural domains against the Pfam database [55] . Particular attention was paid to breakpoints that occurred outside of structural domains of the kinase and the fusion protein partner. Fusion partner sequences were checked for presence of CC domains by the method of Lupas et al. [56] Other dimerization or multimerization domains were checked within partner protein sequences using InterPro [57] . RNA-seq expression quantification mRNA gene expression, measured in fragments per kilobase of mRNA per million mapped reads, were calculated for all CCDS transcripts [58] in the Gencode v17 database [51] using Cufflinks v2.1.1 (ref. 59 ) with the options that included the following: cufflinks --multi-read-correct, --GTF <gencode.annotation.CCDS.gtf>, --mask-file <gencode.annotation_chrM.gtf> <Aligned.bam>. Copy number data Copy number data were downloaded from the 2014-04-16 release on the GDAC portal ( http://gdac.broadinstitute.org/ ). How to cite this article : Stransky, N. et al. The landscape of kinase fusions in cancer. Nat. Commun. 5:4846 doi: 10.1038/ncomms5846 (2014).